Protein sliding and DNA denaturation are essential for DNA organization by human mitochondrial transcription factor A Mitochondria organize their genome in protein–DNA complexes called nucleoids. The mitochondrial transcription factor A (TFAM), a protein that regulates mitochondrial transcription, is abundant in these nucleoids. TFAM is believed to be essential for mitochondrial DNA compaction, yet the exact mechanism has not been resolved. Here we use a combination of single-molecule manipulation and fluorescence microscopy to show the nonspecific DNA-binding dynamics and compaction by TFAM. We observe that single TFAM proteins diffuse extensively over DNA (sliding) and, by collisions, form patches on DNA in a cooperative manner. Moreover, we demonstrate that TFAM induces compaction by changing the flexibility of the DNA, which can be explained by local denaturation of the DNA (melting). Both sliding of TFAM and DNA melting are also necessary characteristics for effective, specific transcription regulation by TFAM. This apparent connection between transcription and DNA organization clarifies how TFAM can accomplish two complementary roles in the mitochondrial nucleoid at the same time. Human mitochondrial DNA (mtDNA) is a 16.6-kb circular double-stranded DNA (dsDNA) molecule present in thousands of copies in the cell's mitochondrial network. It encodes 13 proteins of the respiratory chain, as well as 2 ribosomal RNAs and 22 tRNAs. Mutations in the mitochondrial genome can cause profound problems that are linked to a variety of multisystem disorders [1] . Similar to chromosomal DNA, which is organized into a highly condensed structure to fit within the limited volume of the nucleus, multiple mtDNA molecules are organized into small (~70 nm) protein–DNA complexes called nucleoids [2] , [3] . In eukaryotes, compaction is mostly achieved by wrapping DNA around histones to form nucleosomes. In bacteria, this is accomplished by a combination of mechanisms, including molecular crowding, supercoiling and the action of architectural proteins that bend, wrap or bridge DNA [4] , [5] . To date, little is known about the organization of the mtDNA in mitochondrial nucleoids. Various constituents of the mitochondrial nucleoid have been identified by immunoprecipitation, most of them being involved in essential processes such as mtDNA replication, transcription and repair [6] . The major protein component of the nucleoid is the mitochondrial transcription factor A [7] (TFAM), which is essential for the maintenance of mtDNA and has been implicated in multiple functions in mtDNA metabolism. TFAM was first identified as a transcription factor that binds specifically to the promoter region of the mtDNA and, together with the transcription factor B2, enhances transcription by the mitochondrial RNA polymerase [8] , [9] . The structure of TFAM bound to the promoter region of mtDNA has been solved recently [10] , [11] . It reveals that each of the two high-mobility group (HMG) box domains of TFAM causes the DNA to bend nearly 90°, resulting in a complete U-turn, a favourable arrangement for transcription initiation. TFAM has also been proposed to have an essential role in the organization of the mitochondrial genome [12] , because it shows strong non-sequence-specific DNA binding and is abundant enough to coat the entire mtDNA [13] . Moreover, fluorescence resonance energy transfer and atomic force microscopy (AFM) data suggest that nonspecifically bound TFAM and its yeast homologue, Abf2p, can compact DNA by bending the DNA backbone [10] , [14] and/or promoting the formation of loops [15] , [16] . However, a clear understanding of the assembly of TFAM on mtDNA and the subsequent organization mechanism is lacking. In this study, we characterize the nonspecific DNA assembly dynamics of TFAM, as well as the structural role of TFAM in DNA organization, using a combination of single-molecule manipulation and visualization techniques. We show that TFAM induces compaction by modifying the flexibility of the DNA. Moreover, we observe in real time that TFAM forms highly stable protein patches on DNA, due to the propensity of TFAM to extensively diffuse on DNA before it cooperatively binds on collision with a TFAM patch. On the basis of these observations and, in line with previously reported results [10] , [14] , we propose a molecular mechanism to explain the role of TFAM in DNA organization. TFAM compacts DNA by increasing its flexibility To investigate the interaction of TFAM with nonspecific DNA molecules under different buffer conditions, we performed tethered particle motion (TPM) experiments [17] ( Fig. 1 ). We recorded the root-mean-square (r.m.s.) motion of the beads over time. After addition of TFAM, we observed a lower r.m.s. value, reflecting a decrease in the end-to-end length of the DNA tethers, that is, compaction ( Fig. 1a ). To examine the ionic-strength dependency of this phenomenon, the TPM experiments were performed at different NaCl and MgCl 2 concentrations ( Supplementary Fig. S1 ). A stable reduction of the tether length was observed in buffers with low ionic strength (for example, 75 mM NaCl and 0 mM MgCl 2 ). Under these experimental conditions, TFAM caused a gradual decrease of the r.m.s. value, from 137.9±0.6 nm for bare DNA molecules to 89.3±0.9 nm at saturating TFAM concentration (mean±s.e., N =20; Fig. 1b ). From these experiments, we conclude that TFAM can compact DNA, consistent with its presumed role in nucleoid formation. 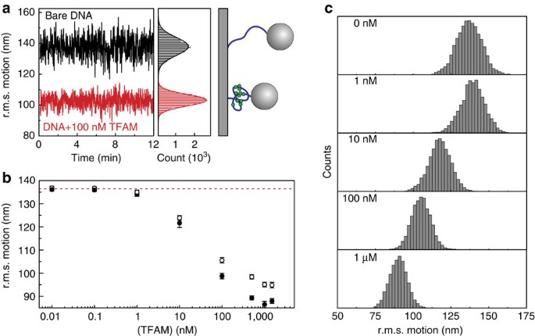Figure 1: TFAM compacts DNA. (a) Typical TPM data traces showing the DNA end-to-end length shortening by TFAM. The root-mean-square (r.m.s.) amplitude of the Brownian motion of the beads is plotted versus time, in the absence (black trace) and presence (red trace) of 100 nM TFAM. The histograms of the r.m.s. motion are shown on the right. The schematic represents a TPM assay: a single DNA molecule is attached between a glass surface and a bead. The amplitude of the restricted Brownian motion of the bead is related to the end-to-end length of the DNA. In the presence of TFAM (green dots) the DNA becomes shorter. (b) Effect of increasing concentration of wild-type TFAM (black symbols) or ΔC-TFAM (open symbols) on the length of DNA (mean±s.e.,N=20). (c) Histograms of r.m.s. motion in the presence of increasing concentration of TFAM. Shown are the r.m.s. motion of DNA tethers with increasing amount of TFAM. The single, well-defined Gaussian distribution of the r.m.s. motion for each of the concentrations indicates that TFAM compacts DNA in the absence of looping. Figure 1: TFAM compacts DNA. ( a ) Typical TPM data traces showing the DNA end-to-end length shortening by TFAM. The root-mean-square (r.m.s.) amplitude of the Brownian motion of the beads is plotted versus time, in the absence (black trace) and presence (red trace) of 100 nM TFAM. The histograms of the r.m.s. motion are shown on the right. The schematic represents a TPM assay: a single DNA molecule is attached between a glass surface and a bead. The amplitude of the restricted Brownian motion of the bead is related to the end-to-end length of the DNA. In the presence of TFAM (green dots) the DNA becomes shorter. ( b ) Effect of increasing concentration of wild-type TFAM (black symbols) or ΔC-TFAM (open symbols) on the length of DNA (mean±s.e., N =20). ( c ) Histograms of r.m.s. motion in the presence of increasing concentration of TFAM. Shown are the r.m.s. motion of DNA tethers with increasing amount of TFAM. The single, well-defined Gaussian distribution of the r.m.s. motion for each of the concentrations indicates that TFAM compacts DNA in the absence of looping. Full size image It has been suggested that, besides having an essential role in the promoter-specific initiation of transcription, the basic C-terminal tail of TFAM is important for nonspecific DNA binding [18] , [19] . To test this, we used a truncated version of TFAM lacking the C-terminal domain (ΔC-TFAM) and monitored the r.m.s. motion of the beads at increasing protein concentrations ( Fig. 1b ). We observed that the truncated protein retained the ability to compact DNA, albeit to a slightly lesser extent than wild-type (WT) TFAM. Hence the C-terminal domain of TFAM is not necessary for the protein to compact DNA. Does this compaction arise from loop formation, as suggested in previous AFM studies [15] , [16] ? In that case, on nonspecific DNA, one would expect that, at each TFAM concentration, loops of varying sizes were formed. In TPM, this would result in a broad distribution of r.m.s. levels, and thus a very broad r.m.s. histogram, as was observed for other looping proteins [17] . In contrast, we observed one well-defined, reproducible, narrow Gaussian distribution at each TFAM concentration ( Fig. 1c ). This indicates that it is unlikely that compaction takes place by unspecific loop formation. To understand how TFAM can compact DNA without forming loops, we used optical tweezers to investigate the elastic properties of bare DNA and TFAM-coated DNA. Single DNA molecules of 48 kb (λ-phage DNA) were end-labelled with biotin and attached between two streptavidin-coated beads [20] ( Fig. 2a ). After capture, the DNA molecules were progressively stretched while the force was measured as a function of DNA extension. A typical force-extension curve of a bare DNA molecule is shown in Fig. 2b . On addition of TFAM, we observed that the mechanical response of the DNA changed significantly. We quantified the TFAM-induced changes of DNA by fitting the force-extension curves with the extensible and the twistable worm-like chain models (including forces of up to 30 and 60 pN, respectively) [21] , [22] . The persistence length ( L p , a measure for the stiffness of the DNA), the contour length ( L c , the total length of the DNA molecule along the backbone), the stretching modulus ( K 0, the spring constant of the DNA backbone) and the twist–stretch coupling of DNA (described by the three parameters g 0 , g 1 and F c ) were obtained for TFAM concentrations ranging from 0.01 to 100 nM ( Fig. 2c ; Supplementary Table S1 ). The values of the DNA's stretching modulus and twist–stretch coupling did not change on addition of TFAM, indicating that TFAM does not modify either the spring constant or the twist–stretch behaviour of the DNA. For the persistence length, we measured a remarkable decrease, from 45.0±6.8 nm for the bare molecules to 3.9±2 nm at saturating TFAM conditions (mean±s.d., N =13), indicating that the molecule was more flexible. Finally, we resolved a slight but significant increase of the DNA contour length (8%; Supplementary Table S1 ). Thus, it seems that DNA compaction by TFAM is mediated by its ability to strongly increase the flexibility of DNA. 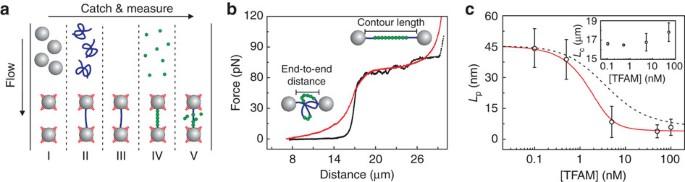Figure 2: TFAM increases the flexibility of DNA and binds to DNA cooperatively. (a) Schematic representation of the multichannel flow cell. Two beads are optically trapped (I); a single DNA molecule is captured between the beads (II); the DNA molecule is moved to a buffer channel where a force-extension curve of the DNA is measured (III); the DNA molecule is incubated with the TFAM protein (IV) and a second force-extension curve is measured in the buffer channel (V). (b) Typical force-extension curve for DNA in the absence (black trace) and presence (red trace) of 50 nM TFAM. The contour length (Lc) and the end-to-end distance of a DNA molecule are schematically depicted. (c) Effect of increasing TFAM concentrations on the persistence length and contour length of DNA (inset; mean±s.d.,N=15). The red line represents the Mc-Ghee-von Hippel fit to our data and the dashed line the Mc-Ghee-von Hippel fit assuming a cooperativity factor of 1. Figure 2: TFAM increases the flexibility of DNA and binds to DNA cooperatively. ( a ) Schematic representation of the multichannel flow cell. Two beads are optically trapped (I); a single DNA molecule is captured between the beads (II); the DNA molecule is moved to a buffer channel where a force-extension curve of the DNA is measured (III); the DNA molecule is incubated with the TFAM protein (IV) and a second force-extension curve is measured in the buffer channel (V). ( b ) Typical force-extension curve for DNA in the absence (black trace) and presence (red trace) of 50 nM TFAM. The contour length ( L c ) and the end-to-end distance of a DNA molecule are schematically depicted. ( c ) Effect of increasing TFAM concentrations on the persistence length and contour length of DNA (inset; mean±s.d., N =15). The red line represents the Mc-Ghee-von Hippel fit to our data and the dashed line the Mc-Ghee-von Hippel fit assuming a cooperativity factor of 1. Full size image Assembly of TFAM nucleoprotein structures Next, we studied how TFAM assembles into compact nucleoprotein structures. We started this investigation by determining the footprint of a single TFAM molecule on DNA, using a combination of optical tweezers and fluorescence microscopy. The fluorescence intensity of single Alexa-555-labelled TFAM monomers was quantified using photobleaching ( Fig. 3a,b ). Thereafter, we determined the total fluorescence intensity of a fully TFAM-coated DNA molecule ( Fig. 3a ) and converted this intensity to the number of TFAM monomers. This way, we found that the footprint of a TFAM monomer was 30.3±0.3 bp (mean±s.e., N =23). To verify this result, we performed a micrococcal nuclease protection assay, which has been used previously to determine the periodic DNA binding pattern of nucleosomes on chromosomal DNA [23] . Radio-labelled DNA of ~500 bp was treated with micrococcal nuclease in the absence or presence of TFAM. After nuclease treatment, an undigested fragment of ~27 bp was observed in the reaction containing TFAM, corresponding to the size of the DNA fragments protected by TFAM ( Fig. 3c ). Another protected fragment of about 10–15 bp could also be observed; however, this fragment was also visible in the control experiment performed in the absence of TFAM, showing that this protected fragment is protein-independent. The size of this footprint confirms the relatively large value determined with our single-molecule assay, and is in agreement with the recently published structural data showing that TFAM makes extensive contact with the DNA [10] , [11] . 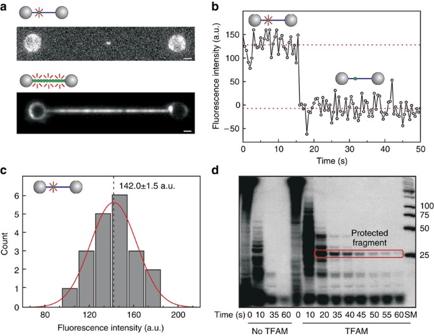Figure 3: TFAM has a footprint of 30 bp on DNA. (a) A single fluorescent TFAM bound to a DNA molecule (upper image) and a DNA molecule fully coated with TFAM (100 nM; lower image). The DNA, held between two beads in the optical tweezers, is not visible. Scale bar, 1 μm. (b) Fluorescence signal of a TFAM–Alexa-555 complex as a function of time, showing a single-step photobleaching event characteristic of a single molecule. (c) Intensity histogram of single TFAM–Alexa-555 complexes. The fluorescence intensity was measured for 20 single complexes and the intensity distribution was fitted with a Gaussian, yielding a mean fluorescence value for a single TFAM–Alexa-555 complex of 142.0±1.5 a.u. (mean±s.e.,N=20). (d) Micrococcal nuclease protection assay. A radioactively labelled DNA fragment was digested with micrococcal nuclease for increasing periods of time in the absence or presence of a constant amount of TFAM. An undigested fragment of approximately 27 bp was obtained. SM, size marker (in bp). Figure 3: TFAM has a footprint of 30 bp on DNA. ( a ) A single fluorescent TFAM bound to a DNA molecule (upper image) and a DNA molecule fully coated with TFAM (100 nM; lower image). The DNA, held between two beads in the optical tweezers, is not visible. Scale bar, 1 μm. ( b ) Fluorescence signal of a TFAM–Alexa-555 complex as a function of time, showing a single-step photobleaching event characteristic of a single molecule. ( c ) Intensity histogram of single TFAM–Alexa-555 complexes. The fluorescence intensity was measured for 20 single complexes and the intensity distribution was fitted with a Gaussian, yielding a mean fluorescence value for a single TFAM–Alexa-555 complex of 142.0±1.5 a.u. (mean±s.e., N =20). ( d ) Micrococcal nuclease protection assay. A radioactively labelled DNA fragment was digested with micrococcal nuclease for increasing periods of time in the absence or presence of a constant amount of TFAM. An undigested fragment of approximately 27 bp was obtained. SM, size marker (in bp). Full size image We analysed the oligomeric state of TFAM bound to DNA, as it has been suggested that TFAM binds in a dimeric form [24] . We used a low concentration of fluorescently labelled TFAM and monitored in real time at the single-protein level the nonspecific TFAM binding to DNA. In this experiment, we always observed the fluorescence disappearing in one step, pointing towards a monomeric state of TFAM on DNA. However, we cannot exclude that this phenomenon is due to dissociation of the protein from DNA. To clarify this point, we compared the average fluorescence intensity of a protein binding event to DNA (57±3 arbitrary unit (a.u.) averaged over the first three frames; mean±s.e. ; N =66) to the value of the fluorescence intensity of a single Alexa-555 (mean±s.e. : 61±2 a.u. ; N =75) and to the value of a single TFAM–Alexa-555 (mean±s.e. : 63±2 a.u. ; N =75) attached to a glass coverslip. These three values were similar, indicating that TFAM binds to DNA from solution as a monomer. Notably, recent crystal structures showed that specific DNA binding of TFAM also happens in a monomeric manner [10] , [11] . When performing these experiments, we discovered that the single TFAM monomers that bind to the DNA nonspecifically started to move rapidly back and forth along the DNA over distances that span several kilobases ( Fig. 4a ; Supplementary Movie 1 ). The movement of TFAM on DNA was tracked with nanometre precision by fitting a two-dimensional Gaussian to the intensity profile in each frame [25] ( Fig. 4b ). Analysis of the motion of TFAM on DNA revealed a linear mean-squared-displacement (MSD; Fig. 4c ), as expected for a protein moving on DNA by one-dimensional diffusion [25] , [26] . The diffusion coefficient obtained from the linear fit was D =(8.6) 10 4 ±0.5 nm 2 s −1 at 25 mM NaCl (mean±s.e., N =66). Proteins use different mechanisms to move along DNA, such as hopping, jumping or sliding [26] . We measured the diffusion coefficient of TFAM over a range of salt concentrations and found that it was not salt-dependent ( D =(9.1±0.7)·10 4 nm 2 s −1 at 75 mM NaCl, N =44, and (7.4±0.9)·10 4 nm 2 s −1 at 150 mM NaCl, N =37), consistent with a sliding mechanism [26] , [27] . 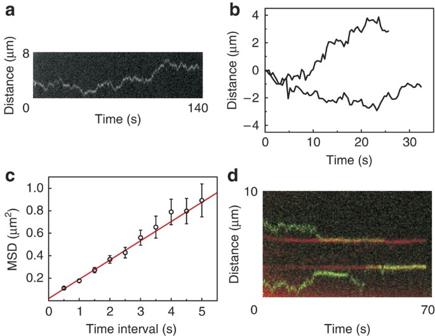Figure 4: Visualizing TFAM diffusion and patches formation on DNA. (a) Kymograph showing the diffusion of TFAM–Alexa-555 on DNA. Time (s) and distance (μm) are indicated at the bottom and left, respectively. (b) Representative trajectories generated from tracking the motion of two single TFAM–Alexa-555. (c) Mean-squared displacement (MSD) of TFAM–Alexa-555 versus time interval (error bars: s.e.,N=66 diffusion traces). The diffusion coefficient is calculated from the linear fit (red line) to the MSD plot. (d) Kymograph showing TFAM patch formation on DNA. TFAM was labelled either with Alexa-555 (green) or Atto-647N (red). The two TFAM preparations were mixed and incubated with the DNA. The fluorescence intensity of a single TFAM–Alexa-555 and a single Atto-647N were determined by single photobleaching steps. On the basis of these values, we determined that the two green moving spots correspond to TFAM monomers, whereas the upper and lower red signals correspond to patches of, respectively, 4 and 6 TFAM molecules. Figure 4: Visualizing TFAM diffusion and patches formation on DNA. ( a ) Kymograph showing the diffusion of TFAM–Alexa-555 on DNA. Time (s) and distance (μm) are indicated at the bottom and left, respectively. ( b ) Representative trajectories generated from tracking the motion of two single TFAM–Alexa-555. ( c ) Mean-squared displacement (MSD) of TFAM–Alexa-555 versus time interval (error bars: s.e., N =66 diffusion traces). The diffusion coefficient is calculated from the linear fit (red line) to the MSD plot. ( d ) Kymograph showing TFAM patch formation on DNA. TFAM was labelled either with Alexa-555 (green) or Atto-647N (red). The two TFAM preparations were mixed and incubated with the DNA. The fluorescence intensity of a single TFAM–Alexa-555 and a single Atto-647N were determined by single photobleaching steps. On the basis of these values, we determined that the two green moving spots correspond to TFAM monomers, whereas the upper and lower red signals correspond to patches of, respectively, 4 and 6 TFAM molecules. Full size image To obtain information on the assembly of TFAM into nucleoprotein structures, we performed a dual-colour fluorescence experiment. To this end, we labelled TFAM with two different dyes, Alexa-555 and Atto-647N, mixed them and visualized their behaviour on DNA ( Fig. 4d ). The fluorescence intensity of single Alexa-555 and Atto-647N-labelled TFAM monomers was quantified using photobleaching ( Supplementary Fig. S2 ). In these dual-colour experiments, we observed that TFAM monomers (and occasionally dimers) diffused along the DNA, while higher-order multimers formed immobile patches. Moreover, when a diffusing TFAM protein encountered a stationary TFAM patch, the diffusion stopped and the protein aggregated with this patch ( Fig. 4d ). Our direct visualization of the assembly of TFAM nucleoprotein structures shows that nonspecific TFAM interaction leads to stable DNA compaction in a two-step mechanism: TFAM monomers first slide on DNA, before assembling into nucleoprotein filaments, by fusing with any encountered patch. Dynamics of TFAM nucleoprotein assembly To further investigate the binding parameters of TFAM on DNA, we incubated DNA molecules with a relatively high concentration of fluorescent TFAM (50 nM). We noticed that DNA molecules incubated for 30 s and imaged in a protein-free region of our microfluidic flow chamber were not uniformly coated. Instead, patches were formed ( Fig. 5a ), as was also observed at lower TFAM concentration ( Fig. 4d ). This observation, together with the sharp decrease of the DNA's persistence length as a function of TFAM concentration ( Fig. 2c ), indicates that TFAM binds to DNA in a cooperative manner. To quantify the cooperative binding of TFAM to DNA, we fitted the concentration dependence of the persistence length with the McGhee-von Hippel model [28] ( Supplementary Fig. S3 ). In this model, the binding of a protein to DNA is characterized by an equilibrium binding constant K (in M −1 ), a cooperativity factor ω and a footprint n . Using our previously obtained footprint of TFAM on DNA as a fixed parameter, the fit yielded a cooperativity factor ω of 70±40. This implies that TFAM is ~100 times more likely to stably bind next to an already bound TFAM than to bare DNA. The fit also yielded an equilibrium binding constant K between 0.9×10 6 and 2.4×10 6 M −1 (best fit: K =1.6×10 6 M −1 ), which corresponds to a value of 1/K of approximately 6×10 −7 M ( Fig. 2c ). This value is within the range of affinities reported earlier for TFAM (approximately 0.6×10 −7 M) [15] , [19] and the (low) affinity of the yeast homologue Abf2p (approximately 25×10 −7 M) [16] , [29] . The difference between our numbers and the reported ones is likely due to a combination of different factors, such as the length of the DNA used and the ionic strength. 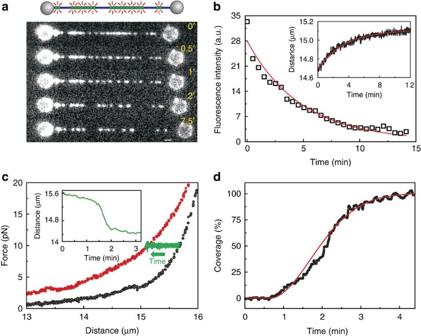Figure 5: Unbinding and binding dynamics of TFAM on DNA. (a) Selected frames from a movie recording the unbinding of TFAM from DNA. Scale bar, 1 μm. (b) Intensity trace of a single DNA molecule covered with TFAM held at constant tension (open square symbols). The data were fit as described in the Methods section (red line). The distance between the two beads (inset) increases as the fluorescence intensity decreases. (c) Real-time association of TFAM to a single DNA molecule. A force-extension curve was measured before (black symbols) and after (red symbols) incubation of the DNA molecule with 50 nM TFAM. During incubation, the DNA molecule was held at constant tension (10 pN) and the distance between the beads was recorded over time (green symbols and inset). (d) The distance measured incwas converted to a percentage of protein coverage and plotted versus incubation time (black symbols). The experimental data points were fitted with a Monte-Carlo simulation (Methods; red trace). Figure 5: Unbinding and binding dynamics of TFAM on DNA. ( a ) Selected frames from a movie recording the unbinding of TFAM from DNA. Scale bar, 1 μm. ( b ) Intensity trace of a single DNA molecule covered with TFAM held at constant tension (open square symbols). The data were fit as described in the Methods section (red line). The distance between the two beads (inset) increases as the fluorescence intensity decreases. ( c ) Real-time association of TFAM to a single DNA molecule. A force-extension curve was measured before (black symbols) and after (red symbols) incubation of the DNA molecule with 50 nM TFAM. During incubation, the DNA molecule was held at constant tension (10 pN) and the distance between the beads was recorded over time (green symbols and inset). ( d ) The distance measured in c was converted to a percentage of protein coverage and plotted versus incubation time (black symbols). The experimental data points were fitted with a Monte-Carlo simulation (Methods; red trace). Full size image Direct visualization of TFAM binding at high concentrations is impossible because of the fluorescent background in the protein channel of our microfluidic flow chamber. However, TFAM binding decreases the persistence length of the DNA, which, in turn, results in a shortening of the end-to-end length of DNA kept under constant tension (10 pN) ( Fig. 5c , green arrow and inset). Therefore, monitoring this change provides a suitable approach to follow TFAM assembly on DNA in real time. We converted the measured DNA end-to-end distance into a fractional coverage of the DNA ( Supplementary Fig. S3 ). The sharp sigmoidal shape of the saturation curve is consistent with a cooperative binding mode ( Fig. 5d , black symbols). We performed Monte Carlo simulations to interpret this saturation curve and to extract the nonspecific TFAM binding rate ( Fig. 6, and Methods section). In this model, we included the observed diffusion and recruitment of TFAM monomers to patches by defining an 'enlarged target site' at the ends of these patches. The enhanced binding at these enlarged target sites is defined by the cooperativity factor we determined previously ( ω ~100; Fig. 6 ). By using these assumptions, we could reproduce and fit our data ( Fig. 5d , red line). This simulation yielded an average association rate per base pair of (3.5±0.5)×10 2 M −1 s −1 per bp (mean±s.d., N =10). The S-shape of the measured curve could only be reproduced by assuming cooperativity for binding, but not by assuming cooperative dissociation. Furthermore, we found an enlarged target size for binding of at least 200 bp. We interpret this enlarged target site as the minimal distance a TFAM monomer scans while diffusing, which is consistent with our diffusion experiments, showing that TFAM is able to diffuse over distances up to several micrometres. 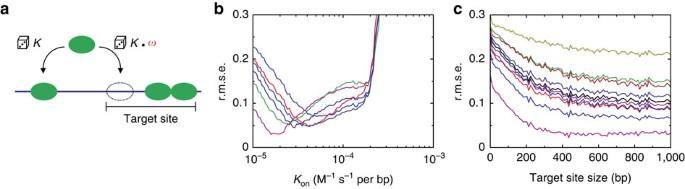Figure 6: Determination of the association rate per site and the enhanced target site of TFAM by Monte-Carlo simulations. (a) One-dimensional lattice of protein binding sites (bp of the DNA). For each time step, there is a certain probabilityKfor a protein to bind to the lattice (left). If, however, there is a protein already bound within a certain distance (enhanced target site), the probability of binding of a new protein is enhanced by a factorω(right). (b,c) Fits of the experimental data to the simulation curves. (b) The r.m.s.e. along theKonaxis ofN=10 traces shows a clear minimum that gives the best fit to our data set. (c) The r.m.s.e. along the target site axis, in contrast, presents a very flat behaviour, indicating that as soon as the target size is around a few hundred base pairs long, increasing its size does not result in a better fit. Figure 6: Determination of the association rate per site and the enhanced target site of TFAM by Monte-Carlo simulations. ( a ) One-dimensional lattice of protein binding sites (bp of the DNA). For each time step, there is a certain probability K for a protein to bind to the lattice (left). If, however, there is a protein already bound within a certain distance (enhanced target site), the probability of binding of a new protein is enhanced by a factor ω (right). ( b , c ) Fits of the experimental data to the simulation curves. ( b ) The r.m.s.e. along the K on axis of N =10 traces shows a clear minimum that gives the best fit to our data set. ( c ) The r.m.s.e. along the target site axis, in contrast, presents a very flat behaviour, indicating that as soon as the target size is around a few hundred base pairs long, increasing its size does not result in a better fit. Full size image Finally, we investigated the unbinding of TFAM from DNA in real time by monitoring the fluorescence intensity of DNA–TFAM complexes ( Fig. 5a ). The decay of intensity allowed a direct measurement of the dissociation time ( Fig. 5b ). Under our experimental conditions (25 mM NaCl, 10 mM Tris, pH 7.6), the dissociation of TFAM was fairly slow: 315±50 s (mean±s.e., N =15), corresponding to a rate of (3.2±0.6)×10 −3 s −1 . The salt dependence of the dissociation was examined by performing the same experiment at increasing monovalent and divalent salt concentrations ( Supplementary Fig. S4 ). We found that the dissociation rate increases with increasing salt concentration, to reach, in more physiological conditions (150 mM NaCl), a rate of (3.0±1.0)×10 −2 s −1 . In this study, we investigated the mechanisms by which TFAM compacts DNA. We show that TFAM is able to bind and compact DNA under tensions up to 40 pN ( Supplementary Fig. S5 ). In contrast, compaction by nucleosomes through wrapping is slowed down at 5 pN, and even inhibited at tensions exceeding 10 pN (ref. 30 ). Furthermore, DNA wrapping results in a shorter DNA molecule [30] , while TFAM actually slightly increases the DNA's length. A wrapping mechanism can therefore be excluded. Similarly, compaction by bridging of DNA molecules, as used by H-NS [5] , [31] , is very improbable, because our TPM experiments show that TFAM does not loop DNA. Moreover, in our optical tweezers experiments, when extending a DNA molecule that had been incubated in a completely relaxed conformation with TFAM, two characteristics of DNA bridging [5] (that is, an effective decrease in the DNA's contour length; and an increase of force, followed by decreases of force as the bridges break on DNA stretching) were not observed. We can thus exclude DNA looping and/or bridging as mechanisms for DNA compaction by TFAM. It should be noted that an increased DNA flexibility due to TFAM binding makes it easier for DNA to coil up on a surface which, in an AFM image, might appear as a looped DNA molecule, as has been reported previously [15] . One hypothesis that can explain DNA compaction is a bending mechanism, in which the protein would introduce multiple bends in the DNA backbone. Several non-sequence-specific architectural proteins, such as the eukaryotic HMG and the non-histone HU bacterial protein [4] , [32] , have been proposed to compact DNA this way. The introduction of such bends would cause an apparent change of the DNA's flexibility, and would thus be consistent with the observed decrease of the DNA's persistence length in the presence of TFAM. AFM and fluorescence resonance energy transfer (FRET) experiments have shown that TFAM and Abf2p decrease the end-to-end distance of DNA [10] , [14] , [16] . This is in agreement with our TPM data where we also measured a decreased DNA end-to-end distance in the presence of TFAM. Some of these articles indicated that the decrease of end-to-end distance would result in the formation of 'rigid' bends in the DNA [15] , [16] . Recent crystallographic analyses of TFAM bound to its specific binding site have shown that the two HMG domains of TFAM lock into the DNA minor groove to generate two 90° kinks, resulting in a U-turn of the DNA [10] , [11] . If such 'rigid' bends would also be introduced by unspecific binding of TFAM to DNA, exerting a force on the DNA would energetically disfavour protein binding and enhance protein dissociation [33] . To test this hypothesis, we measured the dependence of TFAM association and dissociation on the force exerted on the DNA ( Supplementary Fig. S5 ). We found that both association and dissociation of TFAM from DNA were force-independent. Moreover, we noticed that TFAM binding was stable even after multiple cycles of DNA extension/relaxation. In a previous study, we investigated the impact of force on DNA bending [34] and showed that even mild bending would be hampered by tension on the DNA. It is thus unlikely that DNA compaction by TFAM is achieved by the formation of rigid bends in the DNA backbone. It is also possible that TFAM binds and stabilizes spontaneous DNA bends. However, again, TFAM binding would then be slowed down under tension. We instead propose that, in contrast to the ∼ 180° static DNA bend created when TFAM interacts with its specific binding site [10] , [11] , nonspecific binding of TFAM makes DNA more flexible. In fact, small-angle X-ray scattering (SAXS) experiments have shown that TFAM in solution is highly flexible—a flexibility that is conferred by the linker region and the C-terminal domain [11] . The difference between a fixed bend at a specific site, and a broad range of angles at a nonspecific site, could be explained by the fact that, for the specific DNA site at light strand promoter (LSP), there is a fixed optimal distance between the two HMG binding sequences, thus imposing a static bend in the DNA. The compaction mechanism we thus propose is called a 'flexible hinge' model. This model has first been proposed for the architectural proteins HU [4] and HMG [32] . These proteins, similar to TFAM, induce a large decrease of the DNA's persistence length, with little or no change of the contour length. Also, it was shown in an optical tweezers experiment that HMG did not unbind when high forces (up to 150 pN) were applied to the DNA [35] . Thus, our results are most consistently explained by a flexible hinge model, in which the nonspecific DNA binding of TFAM increases the intrinsic flexibility of the DNA, causing the formation of an ensemble of bending angles. Such a 'flexible hinge' model can yield an apparent 'rigid' bending angle, because the calculated bending angle is an average of all the possible angles that can be formed on TFAM binding. This would thus explain the observed 78, 72 and 100±20 degrees angles obtained in previous studies [14] , [15] , [16] , but at the same time provide an explanation for the insensitivity of TFAM binding and unbinding to force. How could TFAM induce DNA flexibility? We noticed in the force-extension curves that the so-called overstretching transition (a region where the DNA lengthens by almost a factor of two at a force of ~65 pN) changes on addition of TFAM ( Fig. 2b ). At low salt concentration, during the overstretching transition, the dsDNA melts and is converted into two single-stranded DNA (ssDNA) strands [36] . The force fluctuations during the overstretching transition for the bare DNA molecule are characteristic of a melting of the DNA molecule via an unpeeling of one of the strands, starting from its extremities or from nicks. In contrast, the overstretching transition in the presence of TFAM is smoother, which could indicate a conversion mode that involves base-pair destabilization that is not initiated at the ends of the molecule or at nicks [21] . On the basis of this observation, it might be that the binding of TFAM to DNA induces some local denaturation of the DNA. Moreover, the crystal structures of specific TFAM binding show unwinding of the DNA extending from the bound HMG boxes [10] , [11] . Thus, TFAM molecules might, on stable binding, induce some denatured or unwound DNA around them ( Fig. 7 ). As ssDNA is much more flexible than dsDNA, TFAM binding would thus result in an increase in the DNA's intrinsic flexibility, and thereby promote DNA compaction. The small increase in the DNA's contour length observed in our stretching experiments is also in agreement with the hypothesis that some denaturation might take place because ssDNA has a larger contour length than dsDNA. 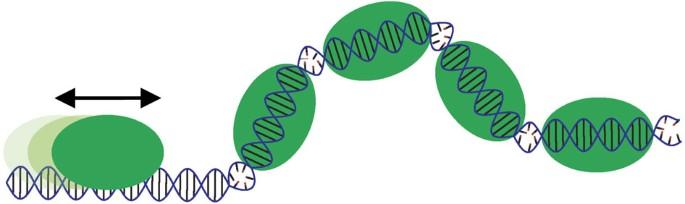Figure 7: Model of cooperative patch formation and DNA compaction by TFAM. TFAM binds to DNA and diffuses until it reaches an already formed patch. This nonspecific DNA binding results in an enhancing of the DNA's intrinsic flexibility, possibly by a local denaturation of the DNA, and thus a compaction of the DNA. This melting of the DNA occurs when TFAM is stably bound to the DNA, not when it is rapidly moving on the DNA. Assuming that this is the mechanism involved, we estimate the number of base pairs ( x ) that are denatured on TFAM binding, using the value of the contour length obtained in the presence of TFAM ( L cTFAM ): Figure 7: Model of cooperative patch formation and DNA compaction by TFAM. TFAM binds to DNA and diffuses until it reaches an already formed patch. This nonspecific DNA binding results in an enhancing of the DNA's intrinsic flexibility, possibly by a local denaturation of the DNA, and thus a compaction of the DNA. This melting of the DNA occurs when TFAM is stably bound to the DNA, not when it is rapidly moving on the DNA. Full size image with L c dsDNA =0.34 nm per bp, L c ssDNA =0.58 nm per bp and L c TFAM =17.4 μm. Solving equation (1) yields a value of x =3.8±0.4 kb converted from dsDNA into ssDNA per DNA molecule. Using our determined footprint of TFAM, this value corresponds to a melting bubble of 2–3 bp between neighbouring TFAM molecules. We have shown that the binding of TFAM is enhanced by the presence of TFAM already bound on the DNA. What are the mechanisms responsible for TFAM (cooperative) binding? Our two-colour experiments show that, after binding to the DNA, TFAM diffuses until it reaches a patch, whereupon it binds stably. Cooperativity is thus due to an enhancement of the binding of diffusing TFAM molecules next to patches. Our Monte-Carlo modelling further confirms this hypothesis, as we demonstrate that TFAM requires an enhanced target size of at least 200 bp to account for the nucleation and subsequent cooperative binding. An explanation for the stable binding of TFAM after it reaches a patch is that, once in the vicinity of an already bound TFAM, the diffusing protein could sense the structural change in the DNA (that is, melting) induced by the bound protein ( Fig. 7 ). This locally destabilized DNA, in turn, might help the stable binding of TFAM to the DNA. The combination of TFAM sliding and melting could thus explain the observed nucleation behaviour and cooperative binding of TFAM. Finally, we propose that these features of TFAM binding—sliding and melting—could also be used by TFAM when acting as a specific transcription factor. First of all, the propensity of TFAM to slide on the DNA before stable binding could facilitate the localization of the specific binding site in the promoter region—similar to the lac repressor, for which the nonspecific DNA binding associated with sliding considerably increases the rate of target location [37] . Secondly, TFAM could locally melt the surrounding DNA when bound to the promoter region, which would permit the mitochondrial RNA polymerase and the transcription factor B2 to bind and transcription to initiate [38] . This connection between transcription initiation and DNA organization would explain how TFAM can accomplish its two complementary roles in the mitochondrial nucleoid simultaneously. TFAM preparation and labelling WT TFAM and the truncated form of TFAM (ΔC-TFAM) were expressed and purified as previously described for WT TFAM [9] . To obtain fluorescent TFAM, the cysteine residues of the protein were labelled with either maleimide Alexa-555 (Molecular Probes) or Atto-647N dye (Sigma-Aldrich). Unreacted dye was removed from the sample with size-exclusion spin-columns (Sephadex G-25, GE Healthcare). The labelling ratio, determined by single-step photobleaching of labelled TFAM molecules immobilized on a glass surface, was one fluorophore per TFAM monomer. The TFAM enzyme preparation used in all experiments was fully active, as determined using a gel-shift assay. All the experiments were done at room temperature (19 °C). DNA substrates The DNA construct used for the TPM experiments (528 bp) was obtained by PCR amplification of the plasmid pSKFokI, a 2,953-bp derivative of pBluescriptSK(–) [39] , using a digoxigenin-modified reverse primer (5′-DIG-CGATTTCGGCCTATTGGTTAAAAAATGAGC-3′) and a biotin-labelled forward primer (5′-BIO-CAGGCTTTACACTTTATGCTTCCGGCTCG-3′). The PCR was purified using the QIAquick PCR purification kit (Qiagen). Lambda DNA (48,502 bp) used for the dual-optical tweezers experiments was biotinylated at the 5′-ends of both strands using Klenow polymerase, as described in ref. 20 . Micrococcal nuclease digestion assay A radiolabelled fragment of 530 bp was generated by PCR amplification of the plasmid pUC18 using the oligonucleotides: 5′-GTAAAACGACGGCCAGTGCCAAGCTTGC-3′ and 5′-CGATTTTTGTGATGCTCGTCAGGGGGG-3′ as primers, in the presence of α- 32 P dCTP. The PCR was purified on a QIA quick spin column (Qiagen). The labelled DNA fragment (2 fmol) was incubated with 200 fmol of TFAM for 20 min at 20 °C in 10 mM Tris–HCl (pH 8.0), 10 mM MgCl 2 , 1 mM dithiothreitol, 0.1 mg ml −1 bovine serum albumin, and 1 mM CaCl 2 in a final volume of 15 μl. Micrococcal nuclease (1.6×10 −4 U, Sigma) was added and the reaction was incubated at 37 °C and quenched by the addition of EDTA (15 mM final concentration) at the times indicated in the figure legend. The samples were treated with 0.5% SDS and 0.2 mg ml −1 proteinase-K for 60 min at 42 °C, and precipitated by addition of 0.6 ml of ice-cold ethanol. The pellets were dissolved in 10 μl H 2 O and 2 μl of gel loading buffer (0.25% bromophenol blue, 0.25% xylene cyanol FF, 15% Ficoll in water) and separated on an 8% native polyacrylamide gel in 1× TBE buffer. The gel was dried before exposure. Tethered particle motion assay DNA molecules were attached between a glass surface and 440-nm polystyrene beads as described in ref. 17 . Flow cell preparation, data acquisition and analysis were performed as previously described [17] . On average, 40 single DNA tethers were measured simultaneously in a buffer containing 10 mM Tris–HCl, pH 7.6, 1 mM dithiothreitol and the salt (NaCl or MgCl 2 ) concentration indicated in the text. Optical trapping and fluorescence microscopy The combined single-molecule fluorescence and optical trapping instrument, as well as the custom-built microfluidic flow system with multiple laminar channels, has been described in detail elsewhere [20] , [36] . Before use, the flow cell was coated with casein (100 μg ml −1 ), to decrease the adsorption of the protein to the glass surface. To reduce photobleaching of the fluorophores, buffers were degassed and kept under nitrogen atmosphere, and 1 mM of the reducing agent dithiothreitol was added. Determination of diffusion coefficients The diffusion of TFAM on DNA was measured using a low concentration of TFAM (≤20 nM). The acquired movies were analysed with a custom-written tracking program (Labview VIEW, National Instruments). Briefly, the position of a moving TFAM–Alexa-555 was obtained from a two-dimensional Gaussian fit to the intensity profile in each frame [25] , [40] . Only traces with a minimal length of 20 frames (10 s) were used. The obtained positions were connected to form a trajectory from which the displacement for the different time intervals was determined. The MSD was calculated by averaging the squared displacement per time interval over all trajectories measured [40] at a given salt concentration. The diffusion constant ( D ) was calculated from the MSD plot (MSD=2 D t +offset). Determination of disassembly times Single Lambda DNA molecules were incubated in the presence of 50 mM of TFAM–Alexa-555 for 30 s. After incubation, the DNA–protein complex was rapidly moved to the buffer channel (to avoid fluorescence background due to the free fluorescent protein), held at constant tension and visualized by stroboscopic illumination of the sample (usually 0.5 s every 30 s) with a 532-nm excitation laser ( Fig. 5a ). The dissociation times ( τ diss ) were determined by fitting the fluorescence intensity traces over time ( Fig. 5b , black symbols) with equation (2) ( Fig. 5b , red trace): where t diss is the total time, t bleach the illumination time and τ bleach the photobleaching time of the fluorophore (obtained for an independent experiment). Monte-Carlo simulation The association rate per site ( K on ) and the enhanced target site of TFAM were determined by performing Monte-Carlo simulations ( Fig. 6 ). A one-dimensional lattice of protein binding sites (bp of the DNA) was simulated ( Fig. 6a ). For each time step d t (with d t chosen sufficiently small), there is a certain probability K for a protein to bind to the lattice (left). If, however, there is a protein already bound within a certain distance (enhanced target site) the probability of binding of a new protein is enhanced by a factor ω (right). Once bound to DNA, the protein diffuses and forms a patch with the already bound proteins. The simulation ends at a given time or when all lattice sites are occupied. The fraction of sites that are occupied is calculated for each time step and gives the simulated curve ( Fig. 5d, red line). The simulations do not include an off-rate for proteins, as we showed that the association is much faster than dissociation ( Fig. 5b versus Fig. 5d ). To fit the simulated traces to our experimental TFAM-association curves, a database consisting of 10,000 simulated traces was built by varying the target site linearly between 1 and 1,000 and the binding probability K on logarithmically between 10 −5 and 10 −3 s −1 . Each trace in the database was obtained by simulating a DNA molecule of 50,000 bp and was averaged over ten individual simulation runs. The traces were shifted with a time offset t 0 to fit against the experimental data, as the binding time of the first TFAM to the DNA can vary. The reduced χ 2 for every trace was recorded; the global minimum and the shape of the well gave the best fit and the confidence band, respectively. How to cite this article: Farge G. et al . Protein sliding and DNA denaturation are essential for DNA organization by human mitochondrial transcription factor A. Nat. Commun. 3:1013 doi: 10.1038/ncomms2001 (2012).